Electrochemical activation of C–H by electron-deficient W2C nanocrystals for simultaneous alkoxylation and hydrogen evolution The activation of C–H bonds is a central challenge in organic chemistry and usually a key step for the retro-synthesis of functional natural products due to the high chemical stability of C–H bonds. Electrochemical methods are a powerful alternative for C–H activation, but this approach usually requires high overpotential and homogeneous mediators. Here, we design electron-deficient W 2 C nanocrystal-based electrodes to boost the heterogeneous activation of C–H bonds under mild conditions via an additive-free, purely heterogeneous electrocatalytic strategy. The electron density of W 2 C nanocrystals is tuned by constructing Schottky heterojunctions with nitrogen-doped carbon support to facilitate the preadsorption and activation of benzylic C–H bonds of ethylbenzene on the W 2 C surface, enabling a high turnover frequency (18.8 h −1 ) at a comparably low work potential (2 V versus SCE). The pronounced electron deficiency of the W 2 C nanocatalysts substantially facilitates the direct deprotonation process to ensure electrode durability without self-oxidation. The efficient oxidation process also boosts the balancing hydrogen production from as-formed protons on the cathode by a factor of 10 compared to an inert reference electrode. The whole process meets the requirements of atomic economy and electric energy utilization in terms of sustainable chemical synthesis. Direct activation of C–H bonds via selective oxidation of hydrocarbons is of great interest for organic hydrocarbons [1] , [2] . As a typical and important transformation path of C–H bonds, selective dehydrogenation of C–H bonds have been widely used for the production of high value-added compounds such as alcohols, and ketones, and ethers [3] , [4] , [5] . However, the relative stability of C( sp 3 )−H bonds adjacent to aromatic rings make C–H activation quite challenging, and either extreme and rather toxic oxidants as chromium or selenium compounds or noble-metal-catalysts (based on rhodium or palladium) at high temperatures have to be applied to obtain acceptable conversions [6] , [7] , [8] . Moreover, the as-formed side product water from the cleavage of C–H bonds via oxydehydrogenation is free of value. As a result, sustainable strategies are highly desirable to further decrease the economic and environmental footprints of C−H activation processes. Electrochemical transformation is recognized as an environmentally friendly method for the production of various functional molecules driven by electricity under mild conditions [9] , [10] , [11] . Pioneering works of electrochemical synthesis using homogeneous catalysts have demonstrated the advantages of this technique for C–H activation [11] , [12] , [13] , which includes selective oxidation [14] , amination [15] , epoxidation [16] , and dehydrogenative coupling reactions [17] . Most of these reactions have a high atom economy and excellent compatibility with flow reactors for continuous synthesis [18] , [19] . The current strategies to boost the transformation of specific substrates mainly rely on the involvement of functional additives [11] , [20] (e.g., organic ligands, bases, and mediators), a high work potential, and/or sacrificial transition metal electrodes [21] , which all will severely limit real-industry applications. Principally, the preparation of cost-effective and active electrode materials is at least as important as the development of a methodology for selective C–H bonds activation [22] , [23] , [24] , [25] , [26] , [27] , [28] , [29] , and only non-targeted, commercial first-generation electrodes (such as carbon rod, platinum, and reticulated vitreous carbon) are applied as the current collectors in electrochemical organic synthesis at the moment. The significant progress reported using well-designed reaction-specified electrodes in improving the catalytic activity for water splitting, nitrogen reduction reactions, and even carbon dioxide reduction reactions [30] , [31] , [32] , [33] further manifests the huge gap between the design of electrode materials and the requirements of sustainable electrochemical organic synthesis. Herein, we present the proof-of-concept application of electron-deficient W 2 C nanocrystal-based electrodes for the highly efficient electrochemical activation of C–H bonds, highlighting the key importance of the modified physicochemical properties of electrode materials in boosting additive-free C–H activation reactions. A nanoheterojunction composed of W 2 C nanocrystals and nitrogen-doped carbons has been rationally designed to control the number of electrons flowing from W 2 C nanocrystals to nitrogen-doped carbons by increasing the doping concentration in the carbon supports to enhance the interfacial Schottky effect. The as-formed electron-deficient W 2 C nanocrystal-based electrode acts as a functional anode to simultaneously facilitate the alkoxylation of ethylbenzene with methanol on the anode and the balancing hydrogen evolution reaction on the cathode. Both the experimental and theoretical results indicate the key role of the electron deficiency of the W 2 C nanocrystals in capturing ethylbenzene on the anode to substantially increase the reaction rates of alkoxylation and hydrogen evolution reaction processes simultaneously and ensure the stability of the anode without scarifying the current collector. Preparation and characterization of W 2 C/N x C The W 2 C/NC catalysts were prepared via a modified nanoconfinement method (Supplementary Fig. 1 ) from a mixture of dicyandiamide and ammonium tungstate, followed by N 2 -protected thermal pyrolysis at high temperatures. The nitrogen contents ( x at.%) of the W 2 C/N x C samples could be tuned from 3.0 via 2.3 to 1.4 at.% (Supplementary Fig. 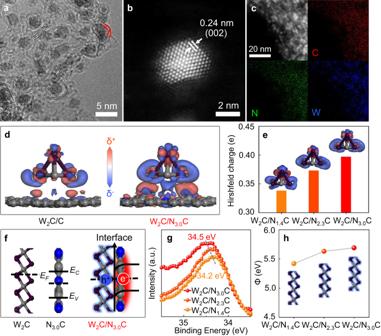Fig. 1: Physical characterizations of the electron-deficient W2C nanocrystals on the NxC. aHigh-resolution TEM image of W2C/N3.0C.bA HAADF-STEM image of W2C/N3.0C.cEnergy-dispersive X-ray elemental mapping of W2C/N3.0C.dElectron density difference stereograms of W2C/C and W2C/N3.0C models (electron-deficient area (δ−), blue; electron-rich area (δ+), red); color code: C, gray; N, blue; W, purple. The small W4C2cluster model represents the W2C nanocrystal.eThe numbers of electrons flowing from W2C nanocrystals to various NxC support models.fSchematic diagrams of the rectifying interface of W2C and N3.0C.gW 4fXPS spectra of W2C/NxC.hWork functions (Φ) of W2C/NxC. 2 and Table 1 ) by elevating the condensation temperatures from 1000 to 1200 °C (for experimental details please see the experimental section). The morphology (Supplementary Fig. 3 ), surface area (Supplementary Fig. 4 ), structure (Supplementary Fig. 5 ), and W content (Supplementary Table 1 ) of W 2 C/N x C samples are well maintained, as reflected by their scanning electron microscopy (SEM) images. Transmission electron microscopy (TEM) observations (Fig. 1a–c and Supplementary Figs. 6 – 8 ) further reveal the presence of few-layer-graphene-supported W 2 C nanocrystals with a mean size of 2.5 nm (Fig. 1a and Supplementary Fig. 9 ) and a typical lattice fringe of 0.24 nm (Fig. 1b ), which corresponds to the (002) plane of α-W 2 C [34] , [35] . The formation of W 2 C is doubly confirmed by its X-ray diffraction (XRD) pattern (Supplementary Fig. 10 ), matching well with that of typical α-W 2 C (JCPDS# 35-776) [34] . Detailed elemental mapping images (Fig. 1c ) exhibit nanometer-sized W-rich areas with a homogeneous distribution of N atoms along with the whole carbon support, indicating an integrated structure of W 2 C nanocrystals on the nitrogen-doped carbons. Fig. 1: Physical characterizations of the electron-deficient W 2 C nanocrystals on the N x C. a High-resolution TEM image of W 2 C/N 3.0 C. b A HAADF-STEM image of W 2 C/N 3.0 C. c Energy-dispersive X-ray elemental mapping of W 2 C/N 3.0 C. d Electron density difference stereograms of W 2 C/C and W 2 C/N 3.0 C models (electron-deficient area (δ − ), blue; electron-rich area (δ + ), red); color code: C, gray; N, blue; W, purple. The small W 4 C 2 cluster model represents the W 2 C nanocrystal. e The numbers of electrons flowing from W 2 C nanocrystals to various N x C support models. f Schematic diagrams of the rectifying interface of W 2 C and N 3.0 C. g W 4 f XPS spectra of W 2 C/N x C. h Work functions (Φ) of W 2 C/N x C. Full size image Identification of electron-deficient W 2 C nanocrystals The highly coupled structure of W 2 C/NC dyads makes it possible to form a rectifying interface for modulation of the electron density of W 2 C nanocrystals. The density functional theory (DFT) calculation results (Supplementary Figs. 11 , 12 ) predict electron transfer from W 2 C to nitrogen-doped carbons, resulting in more pronounced electron-deficient regions in W 2 C nanocrystals suggested by the electron density difference stereograms (Fig. 1d ) of the same W 2 C model supported on pristine carbons (W 2 C/C). The total number of electrons transferred from the small W 4 C 2 cluster to the nitrogen-doped carbon support (Fig. 1e ) increases from 0.338 to 0.397 as more nitrogen atoms (from 1.4 to 3.0 at.%) are doped into the carbon support models (Supplementary Fig. 12j–l ) on the basis of the X-ray photoelectron spectroscopy (XPS) analysis results [36] , while the trend is not affected by the cluster stoichiometry (Supplementary Fig. 13 ). As depicted in Fig. 1f , the nanoheterojunction of W 2 C and NC has a rectifying contact, with electrons flowing from the W 2 C side with a lower Fermi level ( E F ) to the NC side, generating electron-deficient W 2 C due to the interfacial Schottky barrier [37] , [38] . Indeed, the electron donation from the W 2 C nanocrystals to the nitrogen-rich carbon supports is experimentally confirmed by the gradual shift in W 4 f XPS peaks to higher energy (Fig. 1g ) from 34.2 via 34.4 to 34.5 eV for W 2 C/N 1.4 C, W 2 C/N 2.3 C, and W 2 C/N 3.0 C, respectively, resulting in gradually increased work functions (Fig. 1h and Supplementary Fig. 14 ) from 5.4 via 5.6 to 5.7 eV. A similar trend for the electron density of W 2 C nanocrystals in W 2 C/N x C samples is also demonstrated by the most positive W M4,5 peak (Supplementary Fig. 15 ) of the W 2 C/N 3.0 C materials among all samples [39] . All of the above results indicate the formation of electron-deficient W 2 C nanocrystals and the successful further enhancement of electron deficiencies by increasing the nitrogen contents in the carbon supports. Catalytic performance and reaction pathways of catalysts Inspired by the success in modifying the electron density of W 2 C nanocrystals, we further evaluated the possible catalytic activity of W 2 C/N x C catalysts for electrochemical alkoxylation of ethylbenzene with methanol under mild conditions as a model reaction. Considering that the reported methods for alkoxylation of C–H bonds usually require highly active additives/oxidants and/or a high reaction temperature, we initially tested the possibility of additive-free alkoxylation of ethylbenzene with methanol using only a simple electrolyte containing lithium perchlorate and W 2 C/N x C-based electrodes under ambient conditions (Fig. 2 and Supplementary Fig. 16 ). No product was detected without applying a working potential for various electrodes in our electrochemical system (Supplementary Fig. 17a–c ), illustrating that the methoxylation reaction cannot proceed spontaneously. Widely used commercial electrodes, including reticulated vitreous carbon (RVC), boron-doped diamond (BDD), and lead oxide, exhibit poor activity (Supplementary Fig. 17d ) in our additive-free electrocatalytic system. Surprisingly, a complete conversion of ethylbenzene can be achieved on the W 2 C/N 3.0 C electrode with high selectivity to the target product (1-methoxyethyl)benzene (Fig. 2a, b and Supplementary Fig. 18 ) and a total carbon balance of approximately 95%, confirming the possibility of highly efficient alkoxylation of C–H bonds on a well-designed heterogeneous electrode without scarifying additives. The fact that control electrodes with the same amount of bare NC sample, W 2 C catalyst, or a mechanical mixture of the two components (Fig. 2e ) give much lower conversions of ethylbenzene than the W 2 C/N 3.0 C electrode under fixed conditions further indicates a synergistic effect between W 2 C and N 3.0 C components in facilitating the transformation of ethylbenzene. Fig. 2: Catalytic performance of the electron-deficient W 2 C nanocrystal-based anode. a Schematic illustration of electrolyzer and proposed reaction pathway. b The time courses of conversion (red) of ethylbenzene and selectivity (black) to (1-methoxyethyl)benzene on the W 2 C/N 3.0 C anode. c The hydrogen production at the cathode when W 2 C/N 3.0 C and CC were used as the anode. d The time courses of Faradaic efficiencies for conversion of ethylbenzene on the anode and hydrogen production on the cathode, respectively. e Conversions of ethylbenzene on W 2 C/N 3.0 C and control anodes under standard conditions within 3 h. f Cyclic voltammetry curves of typical cathodes (Ti mesh, Pt mesh, and C rod) with the same W 2 C/N 3.0 C anode. Standard reaction conditions: ethylbenzene (0.5 mmol), lithium perchlorate (1 mmol), methanol (15 mL), W 2 C/N 3.0 C anode, and Ti mesh cathode at 2.0 V versus SCE at room temperature in a home-made electrolyzer (Supplementary Fig. 16 ). Full size image Unlike the oxidative alkoxylation reaction of C–H bonds by using various oxidants for dehydrogenation to generate water [40] , our heterogeneous electrochemical system could achieve the full use of as-formed protons from the activation of C–H bonds and methanol for subsequent hydrogen evolution reactions, generating hydrogen gas bubbles on the cathode (Supplementary Fig. 19 and Supplementary Movie 1 ). Moreover, the calculated Faradaic efficiencies (Fig. 2d and Supplementary Fig. 20 ) are similar for the conversion of ethylbenzene to (1-methoxyethyl)benzene on the W 2 C/N 3.0 C anode ( F E : 42–46%) and hydrogen production on the Ti cathode ( F E : 42–55%), implying a cascade transformation of protons generated from the anode into hydrogen gas on the cathode. Even with an excess amount of methanol in the reactor, only a trace amount of formaldehyde (0.006 mmol) formed during the conversion of 0.5 mmol of ethylbenzene (Supplementary Fig. 21 ), well explaining the comparable Faradaic efficiencies for the reactions on anode and cathode without the obvious contribution of methanol dehydrogenation to the total F E for hydrogen evolution reactions. Remarkably, the electron-deficient W 2 C in the W 2 C/N 3.0 C-based electrode substantially promotes the hydrogen evolution rate on the Ti cathode to 880 μmol (Fig. 2c ), which is above 10 times that on the same Ti cathode (85 μmol) when using bare carbon cloth as the anode. The direct release of hydrogen gas on the counter electrode directly confirms the C–H bond activation via single-electron oxidation followed by deprotonation, because as-formed hydrogen atoms from direct hydrogen abstraction could not transfer from W 2 C-based working electrode via the electrolyte solution to the counter electrode for hydrogen gas production. The constant current density of the W 2 C/N 3.0 C anode under fixed conditions with different cathodes (Fig. 2f ), including Pt mesh, Ti mesh, and carbon rod, further demonstrates that the activation of ethylbenzene on the W 2 C/N 3.0 C electrode is the rate dominating step for the whole reaction. The reaction pathways are reasonably proposed via deprotonation of ethylbenzene and followed by methanol addition on the basis of the additional quenching experiments with an additional oxidation peak (Supplementary Fig. 22 ) after the addition of butylated hydroxytoluene (BHT), and no observable signals of any possible radicals were detected, as indicated in Fig. 2 a [41] , [42] . Investigation of the mechanism at heterojunction interfaces The role of the electron-deficient W 2 C nanocrystals and the interfacial effect of the heterojunction catalysts on the electrochemical alkoxylation of C–H bonds were simulated via theoretical calculations and then validated by experimental evidence (Fig. 3 ). The optimized geometry (Fig. 3a, c ) of ethylbenzene presents the preferred adsorption of benzylic C–H bonds on the W 2 C surface dependent on the electron-deficiency of W 2 C, indicating the feature role of W 2 C as an active component. This role was further validated by more negative onset potentials (<1.4 V versus SCE) for the electrochemical alkoxylation reaction on W 2 C/N x C anodes than that (>1.6 V versus SCE) of the bare carbon cloth electrode (Supplementary Fig. 23 ). However, the activation of adsorbed C–H bonds is enhanced by the electron-deficient surface of the W 2 C-0.07e − model, as reflected by the more pronounced electron density difference (Hirshfeld charge) of the preadsorbed C–H bonds (Fig. 3c and Supplementary Fig. 24 ) and a much lower calculated adsorption energy for ethylbenzene (Fig. 3e ). Such strong adsorption of ethylbenzene molecules over the electron-deficient W 2 C surface was then experimentally validated by the temperature-programmed desorption (TPD) analysis results (Fig. 3f ), exhibiting gradually elevated adsorption capacities over those of more electron-deficient W 2 C/N x C samples with similar surface areas. It should be noted that the bare carbon support (NC sample in Fig. 3f ) provides a low adsorption capacity, only 21% of the best-in-class W 2 C/N 3.0 C sample (Supplementary Fig. 25 ). More importantly, the electron deficiency-induced adsorption behavior of ethylbenzene on the final W 2 C/N x C-based anodes under a fixed bias in the electrochemical reactor was well expressed with the same trend in adsorption capacities (Fig. 3g ) as that revealed by TPD results, making successive C–H dissociation process more favorable. Fig. 3: Effect of the electron deficiency of W 2 C nanocrystals on the conversion of ethylbenzene. a , c Electron density difference stereograms of benzylic C–H bonds of ethylbenzene on the surface of W 2 C model ( a ) and electron-deficient W 2 C model (W 2 C-0.07e − ) ( b ). The slice is perpendicular to the plane of benzylic C–H bonds, and electron-rich (red) and electron-deficient (blue) areas are presented. color code: C, gray; N, blue; H, white; W, purple. c , d Calculated absorption configurations of each step of the ethylbenzene activation process on W 2 C ( c ) and W 2 C-0.07e − ( d ). e Gibbs free energy diagrams of each step of the ethylbenzene activation process on W 2 C (black and top) and W 2 C-0.07e − (red and bottom). f Ethylbenzene-TPD results of the W 2 C/N x C and NC samples. g Adsorption capacities of ethylbenzene molecules on the surface of the W 2 C/N x C electrodes with fixed catalyst loadings (0.66 mg/cm 2 ) at 2.0 V versus SCE for 10 min. h Conversions of ethylbenzene on W 2 C/N x C electrodes at 2.0 V versus SCE for 3 h. i Faradaic efficiencies for ethylbenzene conversion on W 2 C/N x C electrodes at 2.0 V versus SCE for 3 h. Full size image Indeed, the stronger interaction between preadsorbed ethylbenzene molecules and electron-deficient W 2 C significantly reduces the Gibbs free energy of each step of the whole alkoxylation reaction pathway (Fig. 3e ). The dissociation of C–H bonds of ethylbenzene on the electron-deficient W 2 C catalyst (W 2 C–0.07e − model) is the rate-limiting step with a free energy change of only 0.34 eV, and the subsequent coupling of *C 8 H 9 and *CH 3 O (*C 8 H 9 + *CH 3 O) and desorption of as-formed (1-methoxyethyl)benzene (*C 9 H 12 O) proceed automatically. With similar configurations, the last three steps for the catalytic conversion of preadsorbed ethylbenzene molecules on the pristine W 2 C catalyst (W 2 C model) are thermodynamically uphill with a larger free energy change of 0.4 eV for the (*C 8 H 9 + *CH 3 O) step, again indicating the key role of electron density in facilitating the whole reaction and desorption processes on the W 2 C surface. This electron-deficiency-dependent promotion effect on the activity of W 2 C was then unambiguously confirmed by the gradually increased catalytic activities (Fig. 3h ) and F E values (Fig. 3i ) for producing (1-methoxyethyl)benzene on more electron-deficient W 2 C/N x C-based anodes under fixed work potential. Stability test and substrate scope The W 2 C/N 3.0 C anode also shows excellent electrochemical stability. The composition (Supplementary Fig. 26 ) and morphology (Supplementary Fig. 27 ) of the used W 2 C/N 3.0 C materials were maintained well. Most importantly, the W 2 C/N 3.0 C anode can be recycled at least four times without an obvious decrease in F E (41−46%) (Fig. 4b and Supplementary Fig. 28 ). It should be noted that inert anodes for alkoxylation of ethylbenzene, including carbon electrode (exemplified by RVC), stable metals (exemplified by Ti mesh), and active metals (exemplified by Ni plate), decompose rapidly within 5 h (Fig. 4a and Supplementary Fig. 29 ), illustrating the key importance of the high activity of the W 2 C/N 3.0 C anode to keep itself from corroding. As the best-in-class anode in this work, the W 2 C/N 3.0 C electrode provides a high turnover frequency (TOF) value of 18.8 h −1 , which is comparable to or even higher than the reported values, mostly of homogeneous catalysts, for similar alkoxylation reactions (Fig. 4c and Supplementary Tables 2 – 4 ) [43] , [44] . Fig. 4: Stability and efficiency of C–H alkoxylation. a Current density change of W 2 C/N 3.0 C, Ti mesh, Ni plate, and RVC electrodes during the reaction. 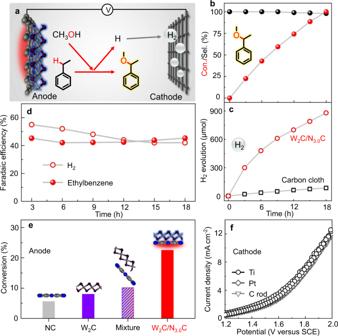Fig. 2: Catalytic performance of the electron-deficient W2C nanocrystal-based anode. aSchematic illustration of electrolyzer and proposed reaction pathway.bThe time courses of conversion (red) of ethylbenzene and selectivity (black) to (1-methoxyethyl)benzene on the W2C/N3.0C anode.cThe hydrogen production at the cathode when W2C/N3.0C and CC were used as the anode.dThe time courses of Faradaic efficiencies for conversion of ethylbenzene on the anode and hydrogen production on the cathode, respectively.eConversions of ethylbenzene on W2C/N3.0C and control anodes under standard conditions within 3 h.fCyclic voltammetry curves of typical cathodes (Ti mesh, Pt mesh, and C rod) with the same W2C/N3.0C anode. Standard reaction conditions: ethylbenzene (0.5 mmol), lithium perchlorate (1 mmol), methanol (15 mL), W2C/N3.0C anode, and Ti mesh cathode at 2.0 V versus SCE at room temperature in a home-made electrolyzer (Supplementary Fig.16). b Reusability of W 2 C/N 3.0 C under standard conditions within 3 h. c TOF values (for details, please see Supplementary Table 2 ) for methoxylation of benzylic C–H bonds on W 2 C/N 3.0 C-based heterogeneous system (solid sphere) and by state-of-the-art photocatalyst (Ir*(III) complex, blue circle) and homogeneous catalyst (CuCl, black circle). Full size image As a durable anode, the electron-deficient W 2 C electrode exhibits satisfying activity for electrochemical alkoxylation of various aromatic C–H bonds using a series of aliphatic alcohols (Fig. 5 ) with good to high conversions and excellent selectivity. Toluene was methoxylated to (methoxymethyl)benzene with high conversion ( 1 ). Benzenes with alkyl chains, including propylbenzene, pentylbenzene, isobutylene, and even halide-substituted substrates ( 2 – 6 ), were successfully transformed into target products with good conversions (20–98%) and very high selectivity (>99%). Alkoxylation of tertiary C–H in cumene ( 7 ) could also proceed smoothly with the alkoxylation product as the sole product. Alkylbenzenes with electron-withdrawing groups ( 8 – 11 ) were also tolerated on the electron-deficient W 2 C-based anode for highly selective alkoxylation reactions even with high steric hindrance. Tetralin and chroman ( 12 and 13 ), as substructures present in numerous drugs, underwent effective methoxylation. It is also not surprising that benzhydryls ( 14 and 15 ) with activated C–H Fig. 5: Scope of substrates catalyzed by W 2 C/N 3.0 C anode. Standard reaction conditions: 1 - 15 , substrate (0.5 mmol), lithium perchlorate (1 mmol), methanol (15 mL), W 2 C/N 3.0 C anode, and Ti mesh cathode with a controlled potential of 2.0 V versus SCE reference electrode for 18 h at room temperature. 16 and 17 , bioactive molecules (0.25 mmol) for 18 h and 4 h, respectively. 18 – 21 , ethylbenzene (0.5 mmol), alcohols (15 mL), W 2 C/N 3.0 C anode, and Ti mesh cathode with a controlled potential of 2.0 V versus SCE reference electrode for 18 h at room temperature. Full size image bonds could be rapidly transformed into alkoxylation products under standard conditions with very high selectivity (>99%). Besides, electrochemical methoxylation could also apply for the late-stage modification of bioactive molecules. 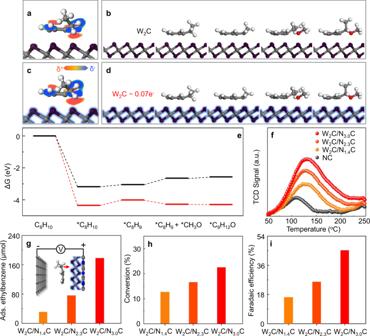Fig. 3: Effect of the electron deficiency of W2C nanocrystals on the conversion of ethylbenzene. a,cElectron density difference stereograms of benzylic C–H bonds of ethylbenzene on the surface of W2C model (a) and electron-deficient W2C model (W2C-0.07e−) (b). The slice is perpendicular to the plane of benzylic C–H bonds, and electron-rich (red) and electron-deficient (blue) areas are presented. color code: C, gray; N, blue; H, white; W, purple.c,dCalculated absorption configurations of each step of the ethylbenzene activation process on W2C (c) and W2C-0.07e−(d).eGibbs free energy diagrams of each step of the ethylbenzene activation process on W2C (black and top) and W2C-0.07e−(red and bottom).fEthylbenzene-TPD results of the W2C/NxC and NC samples.gAdsorption capacities of ethylbenzene molecules on the surface of the W2C/NxC electrodes with fixed catalyst loadings (0.66 mg/cm2) at 2.0 V versus SCE for 10 min.hConversions of ethylbenzene on W2C/NxC electrodes at 2.0 V versus SCE for 3 h.iFaradaic efficiencies for ethylbenzene conversion on W2C/NxC electrodes at 2.0 V versus SCE for 3 h. For example, celestolide ( 16 ) and ibuprofen methyl ester ( 17 ) were able to couple with methanol and shown excellent selectivity at benzylic position. Electron-deficient W 2 C-based anode was also powerful for the alkoxylation of ethylbenzene with different types of aliphatic alcohols ( 18 - 21 ). All these results again reveal the efficiency of the electron-deficient W 2 C catalyst for the benzylic C–H bonds alkoxylation with excellent chemical tolerance to various functional groups. In this work, we have demonstrated the key role of electron-deficient W 2 C nanocrystals as electrode materials in boosting the activity and durability for electrochemical activation of C–H bonds via a heterogeneous pathway. We successfully tuned the electron density of W 2 C nanocrystals by constructing Schottky heterojunctions with nitrogen-doped carbons to achieve preferred adsorption of benzylic C–H bonds of ethylbenzene on the W 2 C surface and facilitate subsequent C–H activation, which is the rate-limiting step. Unlike conventional oxidative alkoxylation to generate water, the as-formed protons on the W 2 C anode could be simultaneously converted to hydrogen gas in our additive-free electrochemical reactor under mild conditions. This two-birds-with-one-stone strategy illustrates the significant potential of powerful designer electrode materials to substantially increase catalytic efficiency, atomic economy, and electric energy utilization for organic electrosynthesis and hydrogen energy production in one electrocatalytic system. In addition to the hydrogen evolution reaction, the reduction process might be compatible with other important reactions (e.g., carbon dioxide reduction reaction or N 2 /NO x reduction reactions) to create more complex cascade reaction pathways for the production of high value-added compounds from abundant hydrocarbons and even waste gases. The electron deficiency shows great potential to enhance the intrinsic activity of catalysts in various catalytic systems, and may also boost the development of zero-additive and zero-emission electrosynthesis systems. We envision that the practical application of the heterojunction-based electrode materials for organic synthesis, commercialized nanocarbons (e.g., nitrogen-doped carbon spheres, carbon nanotube, and even graphenes) could be merged together with functional metal nanoparticles on the surface of various carbon cloth and metal meshes in flow cells for continuous production. Synthesis of W 2 C/N x C All chemicals were analytical grade and used as received without further purification. A homogenous mixed solution including ammonium tungstate ((NH 4 ) 6 H 2 W 12 O 40 ·nH 2 O, 0.75 g), dicyandiamide (DCDA, 15 g), and deionized water (150 mL) was heating at 80 °C, and the mixed solution was evaporated at a constant temperature with stirring. The obtained mixture after evaporating water was transferred into a cylindrical crucible with a lid and heated at 1000, 1100, and 1200 °C for 2 h with a heat rate of 2.5 °C min −1 under a high purity nitrogen atmosphere. The final products after cooling down to room temperature were named W 2 C/N x C ( x represents the nitrogen contents) and used for further experiments and characterizations. The control group of nitrogen-doped carbon (NC) was prepared with the same procedure as W 2 C/N x C without metal precursors. And W 2 C and NC mixture was obtained by mixing W 2 C powder and NC mechanically. Materials characterization Powder X-ray diffraction patterns (XRD) was performed using a Bruker D8 Advance X-ray diffractometer equipped with a Cu Kα radiation source (λ = 1.5418 Å) and operated at a scan rate of 6° min −1 . Scanning electron microscopy (SEM) was operated on FEI Nova NanoSEM 450 field emission scanning electron microscope. Transmission electron microscopy (TEM), high-resolution transmission electron microscopy (HRTEM), and energy-dispersive X-ray (EDX) analysis were measured on a JEM-2100F microscope with an acceleration voltage of 200 kV. Temperature programmed desorption (TPD) was carried out on a Micromeritics Autochem II chemisorption analyzer with ethylbenzene probe molecules at 110 °C. Nitrogen adsorption-desorption isotherms were acquired on Quantachrome NOVA-2200e at 77 K. Prior to the measurement, the samples were degassed at 200 °C for 12 h with a gas flow of nitrogen. X-ray photoelectron spectroscopy (XPS) and ultraviolet photoelectron spectroscopy (UPS) experiments were recorded at a Kratos Axis Ultra DLD spectrometer and ESCALAB 250 photoelectron spectrometer (Thermo Fisher Scientific), respectively. The inductively coupled plasma atomic emission spectroscopy (ICP-AES) measurement was conducted on an iCAP6300 spectrometer for tungsten element analysis. Electrochemical measurements All of the electrochemical experiments were performed in a standard three-electrode system on an electrochemical station (CHI 660E, Shanghai CH Instruments Company). Working electrodes were composed of catalysts supported by carbon cloth. The catalyst ink was prepared by sonicating and dispersing 5 mg of catalyst into a solution containing 700 μL of ethanol, 350 μL of deionized water, and 160 μL of 5% Nafion solution. The working electrodes were prepared by evenly dipping 150 μL of ink onto carbon cloth (1 × 1 cm) and dried at 120 °C for 1 h in the oven. Titanium (Ti) mesh with a size of 1 × 1 cm and saturated calomel electrode (SCE) were employed as counter and reference electrodes, respectively. The control electrodes with different sample loading were prepared by dipping 50, 100, and 200 μL of ink on carbon cloth, respectively. The electrocatalytic reactions were conducted in 15 mL of methanol with 61 μL of ethylbenzene (0.5 mmol) and 0.106 g of lithium perchlorate (1 mmol) at room temperature in a home-made electrolyzer in which methanol was not only used as a solvent but also simultaneously used as a reactant. The electrocatalytic stability tests of catalyst for the reaction between ethylbenzene and methanol were evaluated using the same reaction potential for four consecutive cycles, and electrodes would have to dry at 120 °C before the next reaction. Electrode adsorption experiments were conducted in an electrolyzer containing 1.5 mmol of ethylbenzene, 15 mL of methanol, and 1 mmol of lithium perchlorate with W 2 C/N x C anodes, Ti mesh cathode, and saturated calomel electrode. To accurately measure the adsorption volume of ethylbenzene before transforming (1-methoxyethyl)benzene, we performed at 2 V versus SCE for 10 min. After the completion of adsorption, the residual volume of ethylbenzene in solution was obtained by extraction and analyzed on gas chromatography-mass spectrometry (GC-MS, Shimadzu QP2010SE) with dodecane as internal standard. And the adsorption volume for ethylbenzene on W 2 C/N x C (C ads ) was calculated using the equation of n ads = n ini − n res ( n ini and n res represent the initial and residual contents in solution, respectively) [45] . Products analysis After the reaction, 500 μL of the solution was firstly taken from electrolyzer and transferred into an extracted solution containing 500 μL of dichloromethane, 500 μL of deionized water and 0.2 μL of dodecane, and then dried by magnesium sulfate anhydrous. Finally, the extracted solution was analyzed in GC-MS to determine the components of products and calculate the conversion and selectivity. The Faradaic efficiency ( F E ) was calculated as follow: 
    F_E=N_i×n×F/Q
 (1) where N i is the number of moles for the specific product (mole); n is the number of electrons exchanged for product formation, which is 2 e in this reaction; F is the Faradaic constant of 96487 C mol −1 ; Q is the passed charge. Turnover frequency (TOF) was defined by the following equation: 
    TOF=n/N×h
 (2) where n is the number of moles for the product; N is the number of moles of active metal sites determined from ICP-AES. Theoretical calculation The spin polarization density functional theory (DFT) calculations were performed by the DMol3 program on Materials Studio. The generalized gradient approximation method with Perdew-Burke-Ernzerhof functional (GGA-PBE) was used for describing the exchange-correlation interaction among electrons [46] . The double numerical plus polarization (DNP) basis set was employed, while an accurate DFT semi-core pseudopots (DSPP) was adapted to describe the metal atoms [47] , [48] . The 6 × 6 × 1 k-points were used for sampling the Brillouin zone. 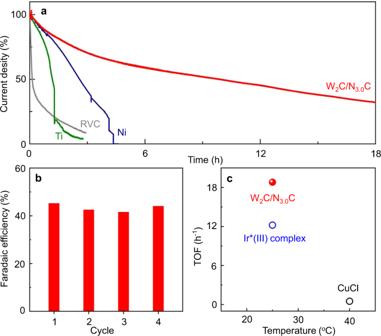Fig. 4: Stability and efficiency of C–H alkoxylation. aCurrent density change of W2C/N3.0C, Ti mesh, Ni plate, and RVC electrodes during the reaction.bReusability of W2C/N3.0C under standard conditions within 3 h.cTOF values (for details, please see Supplementary Table2) for methoxylation of benzylic C–H bonds on W2C/N3.0C-based heterogeneous system (solid sphere) and by state-of-the-art photocatalyst (Ir*(III) complex, blue circle) and homogeneous catalyst (CuCl, black circle). 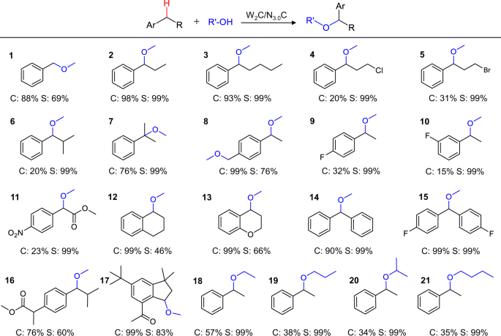Fig. 5: Scope of substrates catalyzed by W2C/N3.0C anode. Standard reaction conditions:1-15, substrate (0.5 mmol), lithium perchlorate (1 mmol), methanol (15 mL), W2C/N3.0C anode, and Ti mesh cathode with a controlled potential of 2.0 V versus SCE reference electrode for 18 h at room temperature.16and17, bioactive molecules (0.25 mmol) for 18 h and 4 h, respectively.18–21, ethylbenzene (0.5 mmol), alcohols (15 mL), W2C/N3.0C anode, and Ti mesh cathode with a controlled potential of 2.0 V versus SCE reference electrode for 18 h at room temperature. Hexagonal W 2 C (002) facets were modeled in terms of the slabs of 5 × 5 supercells with 14.76 × 14.76 Å and 120 o and W 2 C cluster model was placed above a 6 × 6 supercell of graphene lattice [49] . The vacuum slab was set as 20 Å to calculated all periodical models. The structure of the carbon support models was constructed on the basis of concentrations of pyridinic N and graphitic N dopants in the carbon lattice from the XPS analysis results. It should be noted that the bond lengths of small cluster models were fixed during the calculations. The charge exchange was calculated based on a small W 4 C 2 cluster and NC support. The mean number of 0.07 electrons per atom (Supplementary Fig. 12 ) according to the W 4 C 2 cluster/N 3.0 C model was used for following the construction of charged W 2 C slab model to study the interaction between reactant molecule and catalyst surface [50] . It should be noted that the small cluster models are not used for following the simulation of the catalytic process. For the W 2 C slab models, the crystal unit model with the selected (002) facet was used according to HRTEM (Fig. 1b ) and XRD (Supplementary Fig. 10 ) analysis. The Gibbs free energy change (Δ G ) for each step of ethylbenzene activation was calculated as follows: 
    Δ G=Δ E+ΔZPE-TΔ S(T=298.15 K)
 (3) where Δ E , ΔZPE, and Δ S are the changes in the reaction energy, zero-point energy, and entropy, respectively.